PPARγ-induced PARylation promotes local DNA demethylation by production of 5-hydroxymethylcytosine Recent studies have shown that DNA demethylation goes through the conversion of 5-methylcytosine (5mC) to 5-hydroxymethylcytosine (5hmC) by Tet proteins. However, it is still unclear how the target regions for demethylation are distinguished within their genomic context. Here we show that the nuclear receptor peroxisome proliferator-activated receptor-γ (PPARγ) has the ability to direct local demethylation around its binding sites, the PPAR response elements (PPREs), during adipocyte differentiation. PPARγ is a key regulator of the differentiation process that forms a PPARγ co-activator complex on PPREs and activates the expression of adipocyte-specific genes. The complex is poly(ADP-ribosyl)ated (PARylated) on PPREs, and Tet proteins catalyse the conversion of 5mC to 5hmC locally by their ability to bind to the PAR polymer, thereby inducing region-specific demethylation. Our study demonstrates that a sequence-dependent transcription factor complex can, through its post-translational modification, serve for Tet proteins as a landmark to identify sites of DNA demethylation. Methylation of the C5 position of the cytosine base of a CpG dinucleotide, termed DNA methylation, is one of the best characterized epigenetic marks in the mammalian genome [1] . Methylation in promoter/enhancer regions leads to compaction of chromatin, which serves as a transcriptional silencer. Conversely, DNA demethylation induces relaxation of the chromatin and transforms it into a transcriptionally active state [2] . Despite the long-standing understanding of the importance of methylation, the mechanism by which demethylation of 5-methylcytosine (5mC) is processed remains uncertain. Recently, however, studies have suggested that during DNA demethylation, 5mC is converted to 5-hydroxymethylcytosine (5hmC) by Tet proteins, and that 5hmC and following intermediates are replaced by unmodified cytosine [3] . The nuclear receptor peroxisome proliferator-activated receptor-γ (PPARγ) is the key regulatory factor in adipogenesis and directly controls the expression of numerous adipocyte-specific genes, such as adiponectin , aP2 (adipocyte protein 2), Resistin and GLUT4 (glucose transporter 4), by binding to the PPAR-response elements (PPREs) present in the promoter/enhancer regions of these genes [4] . PPARγ is activated in a ligand-dependent manner to switch its binding partner from a co-repressor complex to a co-activator complex on PPREs. Both PPARγ complexes contain various epigenetic molecules such as the histone acetyltransferase p300/CBP [5] , various histone deacetylases [6] , the methyltransferase CARM1 [7] and a SWI/SNF complex, which act as chromatin remodelling factors [8] . These components alter the epigenetic status of the chromatin and regulate expression of adipocyte-specific genes depending on the state of PPARγ. Poly(ADP-ribosyl)ation (PARylation) is a post-translational modification of proteins mediated by poly(ADP-ribose) polymerases (PARPs). PARPs and PARylation have long been studied for their roles in signal transduction in DNA damage and the DNA repair pathway. Recent studies have shown that PARylation is also involved in many other processes such as transcriptional regulation, telomere cohesion and energy metabolism [9] . In addition, it has been suggested that PARylation may have a role in DNA demethylation, particularly in the renewal of 5mC by base excision repair of 5hmC or other intermediates [10] , [11] . Increased PARylation has also been detected during adipocyte differentiation of 3T3-L1 cells; inhibition of PARylation interferes with this differentiation process [12] , [13] . PARPs are also known to be involved in and to modify the PPARγ complex, thereby regulating its transcriptional activities [14] , [15] , [16] . Despite recent advances in research on the mechanism of DNA demethylation, the process by which specific regions within the genome are targeted for demethylation remains uncertain. In this study, we demonstrate that PPARγ promotes the local production of 5hmC around PPREs by recruiting Tet1 through protein PARylation, and thereby induces region-specific demethylation. We find that PPARγ induces DNA demethylation in small regions around PPREs during adipocyte differentiation. The demethylation requires the direct binding of PPARγ and the formation of a co-activator complex on PPREs. Furthermore, we demonstrate that region-specific demethylation involves the production of 5hmC by Tet proteins, and inhibition of PARylation suppresses production of 5hmC. The PPARγ complex on the PPRE is poly(ADP-ribosyl)ated (PARylated), and Tet1/Tet2 locally catalyses hydroxymethylation of 5mC by its ability to bind the PAR polymer. These results demonstrate that the target region of DNA demethylation is determined by PARylation of a sequence-dependent transcription factor complex as a landmark. PPREs of adipose genes are demethylated upon differentiation Most of the genes expressed in adipocytes have functional PPREs on their promoter/enhancer regions, and are regulated by the PPARγ co-repressor/co-activator complex formed on each PPRE. We first analysed the DNA methylation status around the PPREs of some adipose genes in 3T3-L1 cells before and after differentiation by bisulphite sequencing. The adipocyte-specific gene Plin1 has a PPRE 2 kbp upstream of the transcription start site [17] , [18] . Before differentiation, most methylation sites in the Plin1 promoter region were methylated; after differentiation of the cells into adipocytes, these sites were demethylated ( Fig. 1a ). Similar results were obtained from our analyses of the other adipose genes aP2, Resistin , Catalase and PEPCK [19] , [20] , [21] , [22] , [23] , [24] . We observed region-specific demethylation adjacent to the PPREs in these genes similar to that found in Plin1 ( Supplementary Fig. S1 ). 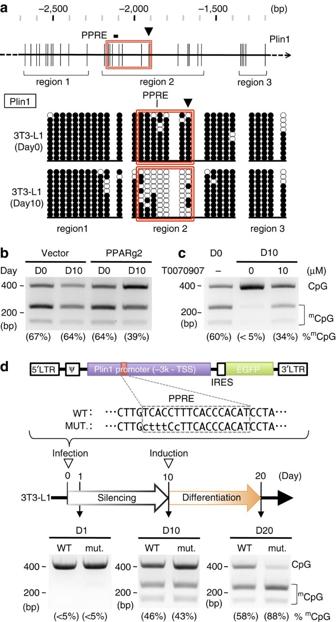Figure 1: PPRE in the enhancer region ofPlin1gene is demethylated during adipocyte differentiation. (a) Bisulphite sequencing analyses of thePlin1promoter. Methylation status of 3T3-L1 cells was analysed before (day 0) and 10 days after (day 10) differentiation induction. At the top of the schematics, the methylation sites around the PPRE are depicted. Vertical lines indicate each CpG. The regions amplified in a string by bisulphite conversion PCR are marked below. At the bottom of the illustrations, the methylation status of the CpGs within each amplified region is shown. Closed circle, methylated; open circle, unmethylated; red boxes, regions with demethylation of >30% of the sites. The CpG indicated by the black triangles is the site assayed in RE assays. (b) Demethylation of thePlin1promoter by overexpression of PPARγ2 in uninduced 3T3-L1 preadipocytes. 3T3-L1 preadipocytes were infected with either empty vector or PPARγ2 expression vector, and were cultured for 10 days. The methylation status of the CpG in thePlin1promoter (the black triangle ina) was evaluated before (D0) and 10 days after (D10) the infection, by its sensitivity to HpyCH4IV (RE assay). The proportion of methylated CpGs (that is, digested fragments) is given below each lane. (c) Inhibition of differentiation-induced demethylation of thePlin1promoter by an antagonist of PPARγ. 3T3-L1 cells were induced to differentiate with or without 10 μM T0070907 for 10 days. Methylation status was measured by RE assay before (D0) and 10 days after (D10) the induction. (d) Methylation analysis of the introduced provirus containing the mutatedPlin1promoter. (Upper) A schematic illustration of the viral vectors containingPlin1promoter with or without mutations in the PPRE. The nucleotide sequences of the PPRE in the vectors are shown below. Dashed rectangle, the PPRE; the small letters indicate the mutated nucleotides. (Middle) Timeline of virus infection and differentiation induction of the 3T3-L1 cells. Methylation of the introducedPlin1promoter was analysed immediately after infection (D0), before differentiation (D10) and after differentiation (D20). (Lower) Methylation analysis of the proviralPlin1promoter at each time point as measured by RE assays. Figure 1: PPRE in the enhancer region of Plin1 gene is demethylated during adipocyte differentiation. ( a ) Bisulphite sequencing analyses of the Plin1 promoter. Methylation status of 3T3-L1 cells was analysed before (day 0) and 10 days after (day 10) differentiation induction. At the top of the schematics, the methylation sites around the PPRE are depicted. Vertical lines indicate each CpG. The regions amplified in a string by bisulphite conversion PCR are marked below. At the bottom of the illustrations, the methylation status of the CpGs within each amplified region is shown. Closed circle, methylated; open circle, unmethylated; red boxes, regions with demethylation of >30% of the sites. The CpG indicated by the black triangles is the site assayed in RE assays. ( b ) Demethylation of the Plin1 promoter by overexpression of PPARγ2 in uninduced 3T3-L1 preadipocytes. 3T3-L1 preadipocytes were infected with either empty vector or PPARγ2 expression vector, and were cultured for 10 days. The methylation status of the CpG in the Plin1 promoter (the black triangle in a ) was evaluated before (D0) and 10 days after (D10) the infection, by its sensitivity to HpyCH4IV (RE assay). The proportion of methylated CpGs (that is, digested fragments) is given below each lane. ( c ) Inhibition of differentiation-induced demethylation of the Plin1 promoter by an antagonist of PPARγ. 3T3-L1 cells were induced to differentiate with or without 10 μM T0070907 for 10 days. Methylation status was measured by RE assay before (D0) and 10 days after (D10) the induction. ( d ) Methylation analysis of the introduced provirus containing the mutated Plin1 promoter. (Upper) A schematic illustration of the viral vectors containing Plin1 promoter with or without mutations in the PPRE. The nucleotide sequences of the PPRE in the vectors are shown below. Dashed rectangle, the PPRE; the small letters indicate the mutated nucleotides. (Middle) Timeline of virus infection and differentiation induction of the 3T3-L1 cells. Methylation of the introduced Plin1 promoter was analysed immediately after infection (D0), before differentiation (D10) and after differentiation (D20). (Lower) Methylation analysis of the proviral Plin1 promoter at each time point as measured by RE assays. Full size image To investigate how these DNA demethylations proceeded during differentiation, we monitored the methylation status of CpGs in the demethylated region of the Plin1 promoter by the efficiency of digestion by a restriction enzyme (RE) assay ( Supplementary Fig. S2 ), and found that it proceeded gradually from day 3 to day 7 of differentiation. The proliferation of 3T3-L1 cells is essentially arrested by day 2 (ref. 25 ), and the result suggests that this demethylation is a replication-independent, active process. The levels of expression of Plin1 and PPARγ also increased concurrently with the demethylation of the PPREs. To confirm the involvement of PPARγ in region-specific demethylation, we analysed the effects of forced expression or inhibition of PPARγ on demethylation. RE assay showed that overexpression of PPARγ in undifferentiated 3T3-L1 preadipocytes induced demethylation around the Plin1 PPRE ( Fig. 1b , Supplementary Fig. S3 ). Similarly, demethylation was found after ectopic expression of PPARγ in NIH/3T3 fibroblasts ( Supplementary Figs S3 and S4 ). Bisulfite-sequencing analyses indicated that PPARγ-induced demethylation in NIH/3T3 cells proceeded in the same manner as the differentiation-induced demethylation in 3T3-L1 cells ( Supplementary Fig. S5 ). These results suggested that expression of PPARγ alone was sufficient to induce PPRE-specific demethylation, even in cell lineages other than adipocytes. On the other hand, treatment with T0070907, which inhibits co-activator complex formation of PPARγ and keeps it in repressive state [26] , suppressed the differentiation-associated demethylation of the Plin1 PPRE ( Fig. 1c ), suggesting that the formation of the PPARγ co-activator complex on PPRE is necessary for the demethylation. Next, we sought to determine whether direct binding of PPARγ to PPREs is necessary for the determination of the demethylation region. Retroviral vectors containing the Plin1 promoter, with or without a mutation in the PPRE that abolishes PPARγ binding ( Fig. 1d and Supplementary Fig. S6 ) [18] , were used to infect 3T3-L1 preadipocytes, and the effect of differentiation on the methylation status of each provirus was monitored at various intervals. Immediately after infection, Plin1 promoters in the provirus were still unmethylated. It has been known that a heterogeneous provirus inserted into a genome is gradually silenced by DNA methylation. The infected cells were cultured for 10 days to allow methylation of the provirus; just under half of each provirus was methylated until day 10. The cells were then induced to differentiate (that is, to express PPARγ) and the effect of the mutation in the PPRE on the methylation status of the introduced provirus was observed after another 10 days of culture. As shown in Fig. 1d , the binding of PPARγ counteracted the silencing of the provirus containing the wild-type PPRE and slowed progression of methylation to 58% at day 20. By contrast, the mutated Plin1 provirus showed no such effect and showed a greater level of methylation compared with the wild-type provirus (88% at day 20, Fig. 1d ). These results indicated that, by binding to PPRE, PPARγ determines the regions to be demethylated. Although only a smaller difference was detected in experiments with NIH/3T3 cells (because of relatively weaker silencing), nevertheless, the same trend was observed ( Supplementary Fig. S6 ). PPARγ promotes Tet protein-mediated hydroxylation of 5mC around PPREs To further investigate the mechanisms of the determination of the regions for DNA demethylation, we examined 5hmC production during demethylation. A dot blot analysis of differentiating adipocytes indicated that the amount of 5hmC increased transiently with a peak around day 5–day 7, and a subsequent decline by day 10 ( Fig. 2a ). Ectopic expression of PPARγ in NIH/3T3 cells also resulted in a global increase in the level of 5hmC, indicating that PPARγ-mediated DNA demethylation involves production of 5hmC ( Fig. 2b ). To confirm that the increase in 5hmC occurred in the demethylated regions around the PPREs, we performed DNA immunoprecipitation of Plin1 and aP2 PPREs using an anti-5hmC antibody from genome fragmented by the REs. The fragments containing demethylated regions around the PPREs derived from the genome of PPARγ-expressing NIH/3T3 cells were selectively pulled down, whereas the upstream control regions and the fragments from non-expressing cells were not ( Fig. 2c ). These results suggest that PPARγ has the ability to promote region-specific production of 5hmC around PPREs. 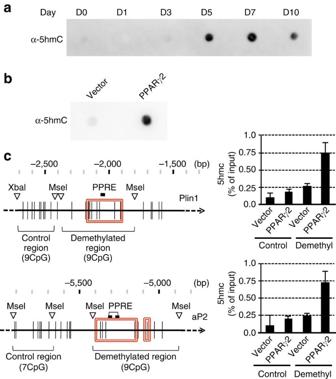Figure 2: PPARγ mediates local 5hmC production around PPREs. (a) Time-lapse analysis of 5hmC by a dot blot during differentiation of 3T3-L1 cells into adipocytes. Total genomic DNA was collected at the indicated time points, and 100 ng of each genome was spotted onto the membrane. (b) Increase in 5hmC after ectopic expression of PPARγ2 in NIH/3T3 cells. Total genomic DNAs were collected 5 days after infection with either PPARγ2 or an empty vector, and 100 ng of each genome was spotted onto the membrane. (c) DNA immunoprecipitation assay of 5hmC around the PPREs ofPlin1andaP2using the genomic DNA used inb. The schematics depict the positions of control and demethylated regions detected by qPCR, and also show the digestion sites of the REs used for fragmentation of each gene. Red boxes indicate regions with demethylation of >30% of the sites (see alsoFig. 1aandSupplementary Fig. S1A). The amounts of control/demethylated regions in the immunoprecipitated DNA and 5% of input were estimated by qPCR and the ratios of the immunoprecipitated to input were presented. (n=3, mean±s.d.). Figure 2: PPARγ mediates local 5hmC production around PPREs. ( a ) Time-lapse analysis of 5hmC by a dot blot during differentiation of 3T3-L1 cells into adipocytes. Total genomic DNA was collected at the indicated time points, and 100 ng of each genome was spotted onto the membrane. ( b ) Increase in 5hmC after ectopic expression of PPARγ2 in NIH/3T3 cells. Total genomic DNAs were collected 5 days after infection with either PPARγ2 or an empty vector, and 100 ng of each genome was spotted onto the membrane. ( c ) DNA immunoprecipitation assay of 5hmC around the PPREs of Plin1 and aP2 using the genomic DNA used in b . The schematics depict the positions of control and demethylated regions detected by qPCR, and also show the digestion sites of the REs used for fragmentation of each gene. Red boxes indicate regions with demethylation of >30% of the sites (see also Fig. 1a and Supplementary Fig. S1A ). The amounts of control/demethylated regions in the immunoprecipitated DNA and 5% of input were estimated by qPCR and the ratios of the immunoprecipitated to input were presented. ( n =3, mean±s.d.). Full size image To date, three members of Tet-family proteins are known as methylcytosine hydroxylation enzyme (Tet1, Tet2 and Tet3), and each protein exhibits different expression patterns by tissues [27] . Western blotting of each Tet proteins in NIH/3T3 and 3T3-L1 cells showed that constant amount of Tet1 and Tet2 were expressed in both cell lines and throughout the differentiation, but Tet3 was slightly expressed ( Supplementary Fig. S7 ). To determine which protein was responsible for the demethylation of PPREs, we performed a knockdown analysis using short-hairpin RNA of Tet proteins [28] . In the differentiating 3T3-L1 cells on day 5, shTet1 showed a certain amount of, and shTet2 showed an apparent decrease of 5hmC. Conversely, a knockdown of Tet3 had slight effect on the amount of 5hmC ( Fig. 3a and Supplementary Fig. S8 ). Knockdown of Tet1/Tet2 in NIH/3T3 expressing exogenously introduced PPARγ2 also repressed the global increase of 5hmC ( Supplementary Fig. S9 ). Knockdown of Tet1/Tet2 in 3T3-L1 preadipocytes interfere with the local demethylation of Plin1 PPRE during differentiation, mRNA expression of Plin1 and aP2, and differentiation to adipocytes ( Supplementary Fig. S10 ). 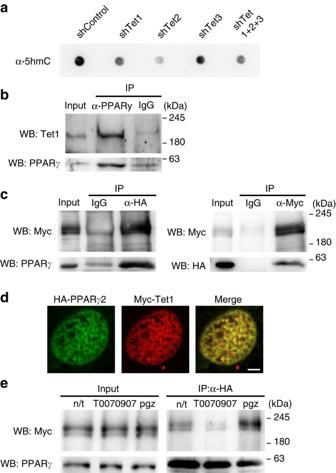Figure 3: Tet1 interacts with PPARγ. (a) Suppression of the increase in 5hmC during adipocyte differentiation by knockdown of Tet proteins. Cells were transfected with the viral short-hairpin RNA (shRNA) vectors 2 days before the induction of differentiation, and total genomic DNAs were collected on day 5 of differentiation. One hundred nanograms of each genome were spotted onto the membrane and detected using anti-5hmC antibody. (b) Interaction between PPARγ and Tet1 in 3T3-L1 cells. PPARγ was immunoprecipitated using anti-PPARγ antibody from a nuclear extract of differentiating 3T3-L1 on day 5. Co-immunoprecipitated Tet1 was detected by western blotting using anti-Tet1 antibody. (c) Interaction between HA-tagged PPARγ and Myc-tagged Tet1. HA-PPARγ2 and Myc-Tet1 were transfected to HEK293 cells and immunoprecipitated using anti-HA/Myc antibody from nuclear extracts of the cells. Co-immunoprecipitated Myc-Tet1/HA-PPARγ2 was detected by western blotting using anti-Myc/PPARγ antibody. (d) Localization of HA-tagged PPARγ2 and Myc-tagged Tet1 in the nucleus of NIH/3T3 cells. A white bar in the merged image indicates 5 μm. (e) Effects of antagonist/agonist of PPARγ on the interaction with Tet1. HA-PPARγ2 and Myc-Tet1 were transfected to HEK293 cells and immunoprecipitated using anti-HA antibody in the presence or absence of 10 μM T0070907 or 10 μM pioglitazone (pgz). Co-immunoprecipitated Myc-Tet1 was detected by western blotting using anti-Myc antibody. Figure 3: Tet1 interacts with PPARγ. ( a ) Suppression of the increase in 5hmC during adipocyte differentiation by knockdown of Tet proteins. Cells were transfected with the viral short-hairpin RNA (shRNA) vectors 2 days before the induction of differentiation, and total genomic DNAs were collected on day 5 of differentiation. One hundred nanograms of each genome were spotted onto the membrane and detected using anti-5hmC antibody. ( b ) Interaction between PPARγ and Tet1 in 3T3-L1 cells. PPARγ was immunoprecipitated using anti-PPARγ antibody from a nuclear extract of differentiating 3T3-L1 on day 5. Co-immunoprecipitated Tet1 was detected by western blotting using anti-Tet1 antibody. ( c ) Interaction between HA-tagged PPARγ and Myc-tagged Tet1. HA-PPARγ2 and Myc-Tet1 were transfected to HEK293 cells and immunoprecipitated using anti-HA/Myc antibody from nuclear extracts of the cells. Co-immunoprecipitated Myc-Tet1/HA-PPARγ2 was detected by western blotting using anti-Myc/PPARγ antibody. ( d ) Localization of HA-tagged PPARγ2 and Myc-tagged Tet1 in the nucleus of NIH/3T3 cells. A white bar in the merged image indicates 5 μm. ( e ) Effects of antagonist/agonist of PPARγ on the interaction with Tet1. HA-PPARγ2 and Myc-Tet1 were transfected to HEK293 cells and immunoprecipitated using anti-HA antibody in the presence or absence of 10 μM T0070907 or 10 μM pioglitazone (pgz). Co-immunoprecipitated Myc-Tet1 was detected by western blotting using anti-Myc antibody. Full size image To examine the interaction of PPARγ with Tet1 and Tet2, we performed co-immunoprecipitation (co-IP) assays using anti-PPARγ antibody and detected the association of Tet1 with PPARγ in a nuclear extract of 3T3-L1 cells on day 5 ( Fig. 3b , Supplementary Fig. S11 ). However, we failed to demonstrate the interaction of Tet2 with PPARγ experimentally, although Tet2 was expressed in a greater amount and seemed to have a larger impact on the increase of 5hmC. The interaction of Tet1 was further confirmed by co-IP assays in HEK293 cells overexpressing Myc-tagged Tet1 and HA-tagged PPARγ2 ( Fig. 3c ). Immunofluorescence analysis also showed that HA-PPARγ2 was co-localized with Myc-Tet1 in the nucleus of NIH/3T3 cells ( Fig. 3d ). We next performed the co-IP assays in the presence of an antagonist (T0070907) or an agonist (pioglitazone) of PPARγ to compare the affinity of Tet1 for co-repressor and co-activator complex formed by PPARγ ( Fig. 3e ). Addition of T0070907 reduced co-IP efficiency of Myc-Tet1 by HA-PPARγ2 compared with no-treatment. In contrast, addition of pioglitazone improved the co-IP efficiency of the no-treatment. These observations indicated that Tet1 exhibited more affinity for co-activator complex formed by a pioglitazone treatment than that for co-repressor complex formed by an addition of T0070907, suggesting that the activation of PPARγ and associated switching from the co-repressor complex to the co-activator complex on PPREs attracts the cytosine hydroxylation enzymes, and thereby causes demethylation of the specified region. The T0070907 treatment showed a reduced co-IP efficiency than the no-treatment sample without affecting enzymatic activity of Tet1 ( Supplementary Fig. S12 ), revealing that the suppression of DNA demethylation by T0070907 observed in Fig. 1c was due to the interference of the recruitment of Tet proteins to the PPRE. PPARγ-induced PARylation mediates region-specific 5hmC production As described in the introduction, increases of protein PARylation are observed on adipocyte-specific genes in 3T3-L1 adipocytes. We also confirmed that the forced expression of PPARγ2 in NIH/3T3 cells increases the global level of PARylation in the nucleus by immunofluorescent microscopy, and also the local PARylation on the PPREs of Plin1 and aP2 by chromatin immunoprecipitation assay ( Supplementary Fig. S13 ). Inhibition of PARylation repressed the increase of Plin1 and aP2 mRNA, and adipocyte differentiation itself ( Supplementary Fig. S14 ). Here we examined the involvement of this protein PARylation in PPARγ-induced demethylation of PPREs. Inhibition of the activity of PARPs by PJ-34 treatment caused a dose-dependent reduction in demethylation of the Plin1 PPRE in PPARγ-expressing NIH/3T3 cells ( Fig. 4a , Supplementary Fig. S15 ), without affecting the amount and the enzymatic activity of Tet1 ( Supplementary Fig. S16 ). As bisulphite conversion analysis does not distinguish 5mC and 5hmC, and exhibits both residues as ‘methylated’, the result suggests that the inhibition of PARylation interferes with the processing of 5mC or 5hmC in the demethylation reaction. A dot blot analysis and a DNA immunoprecipitation assay further showed that inhibition of PARylation suppressed both the global increase in 5hmC in the genome and the local increase around the PPREs driven by PPARγ ( Fig. 4b,c ). These results suggest that protein PARylation is required before the region-specific production of 5hmC. 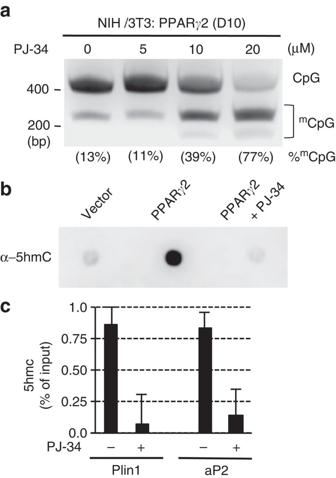Figure 4: Inhibition of PARylation interferes with 5hmC production around PPREs. (a) Effect of PJ-34 treatment on PPARγ-driven DNA demethylation. The methylation status of thePlin1PPRE in NIH/3T3 cells was estimated by an RE digestion assay 10 days after infection with the PPARγ2 vector. (b) Effect of PJ-34 treatment on the global increase in 5hmC induced by PPARγ expression in NIH/3T3. The cells were infected with either PPARγ2 or an empty vector, and were cultured with or without 20 μM PJ-34. Total genomic DNAs were collected 5 days after infection and 100 ng of each genome was spotted onto the membrane. (c) Effect of PJ-34 treatment on the region-specific increase in 5hmC around the PPREs ofPlin1andaP2. The fragmented genomes of PPARγ2-expressing NIH/3T3 cells (5 days after infection, treated with or without 20 μM PJ-34) were immunoprecipitated with an anti-5hmC antibody, and the amounts of the demethylated regions ofPlin1andaP2(indicated inFig. 2c) and 5% of input DNAs were estimated by reverse transcriptase (RT)–PCR. The ratios of the immunoprecipitated to input were presented. (n=3, mean±s.d.). Figure 4: Inhibition of PARylation interferes with 5hmC production around PPREs. ( a ) Effect of PJ-34 treatment on PPARγ-driven DNA demethylation. The methylation status of the Plin1 PPRE in NIH/3T3 cells was estimated by an RE digestion assay 10 days after infection with the PPARγ2 vector. ( b ) Effect of PJ-34 treatment on the global increase in 5hmC induced by PPARγ expression in NIH/3T3. The cells were infected with either PPARγ2 or an empty vector, and were cultured with or without 20 μM PJ-34. Total genomic DNAs were collected 5 days after infection and 100 ng of each genome was spotted onto the membrane. ( c ) Effect of PJ-34 treatment on the region-specific increase in 5hmC around the PPREs of Plin1 and aP2 . The fragmented genomes of PPARγ2-expressing NIH/3T3 cells (5 days after infection, treated with or without 20 μM PJ-34) were immunoprecipitated with an anti-5hmC antibody, and the amounts of the demethylated regions of Plin1 and aP2 (indicated in Fig. 2c ) and 5% of input DNAs were estimated by reverse transcriptase (RT)–PCR. The ratios of the immunoprecipitated to input were presented. ( n =3, mean±s.d.). Full size image To examine whether PARylation mediates the recruitment of Tet1 to PPREs, we compared the subnuclear localization of PPARγ and Tet1 with or without PJ-34 ( Fig. 5a and Supplementary Fig. S17 ). In the absence of PJ-34, PPARγ formed punctate foci in the nucleus and Tet1 was strongly co-localized with them. In the presence of PJ-34, however, Tet1 did not form the foci on PPARγ and diffused throughout the nucleus. Inhibition of PARylation also interfered with co-IP of Tet1 by PPARγ ( Fig. 5b and Supplementary Fig. S18 ). To further examine the binding ability of recombinant Tet1 protein to PAR polymer, we performed PAR-binding assay in vitro ( Fig. 5c ). The membrane-bound Tet1 fragment and histone H1, the positive control, clearly exhibited binding ability to the PAR polymer, but no binding was observed with proteinase K, the negative control. A search for the conserved PAR-binding motif suggested three possible candidates in Tet1 (represented as m1–3 in Fig. 5d ) [29] . To test whether these motifs were functional, we synthesized four peptides that respectively covered the N-terminal region (containing m1; p1), the CXXC zinc-finger domain (p2), the cysteine-rich domain (containing m2 and m3; p3) and the double-stranded beta helix domain (p4) of Tet1, and examined their ability to bind to PAR ( Fig. 5d and Supplementary Fig. S18 ) [30] . We found that peptide p3, which contains m2 and m3, exhibited a strong binding ability, suggesting that Tet1 binds to the PAR polymer by its cysteine-rich domain. Although it was slightly weaker, peptide p1 and p2 also exhibited an ability to bind to PAR. 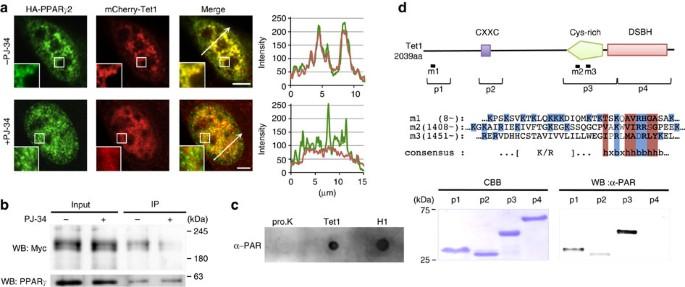Figure 5: PARylation mediates the recruitment of Tet1 to PPREs. (a) Effect of PJ-34 treatment on the localization of HA-PPARγ2 and mCherry-Tet1 in the nucleus of NIH/3T3 cells. The inset left below of each image shows the magnified image of the framed area. The graph at the right of each row indicates the transition of the signal intensity of PPARγ2 (green) and Tet1 (red) along with the white allow in the merged image. White bars in the merged images indicate 5 μm. (b) Effects of inhibition of PARylation on the interaction of PPARγ with Tet1. HA-PPARγ2 and Myc-Tet1 were transfected to HEK293 cells and immunoprecipitated using anti-HA antibody in the presence or absence of 20 μM PJ-34. Immunoprecipitated HA-PPARγ2 and co-immunoprecipitated Myc-Tet1 was detected by western blotting using anti-PPARγ and anti-Myc antibody. (c) PAR-binding assay of Tet1. One microgram of the indicated proteins was dot blotted onto a nitrocellulose membrane and incubated with PAR polymers. Protein-bound polymers were visualized by chemiluminescence with an anti-PAR antibody. pro. K, proteinase K (negative control); Tet1, catalytic domain of Tet1; H1, histone H1 (positive control). (d) PAR-binding motifs in Tet1- and PAR-binding assay of Tet1 peptides. (Upper) The schematic depicts the positions of the three putative PAR-binding motifs (m1–3) and four peptides synthesized for the PAR-binding assay (p1-4) of Tet1. Alignment of the putative PAR-binding motifs with the consensus PAR-binding motif is shown below. A common feature of the motif is the presence of hydrophobic amino acids (h; ACGVILMFYW) spaced by basic amino acids (b; KRH) and an additional accumulation of basic residues at the N-terminal side of the motif. Conserved hydrophobic residues are indicated in bold against a red background, and neighbouring basic amino acids are shown in bold against a blue background. The residues corresponding to the basic block of the N-terminal region are represented against a blue background. (Lower) Images of the peptides dyed by CBB and PAR-binding assay of the peptides transferred onto membrane. Figure 5: PARylation mediates the recruitment of Tet1 to PPREs. ( a ) Effect of PJ-34 treatment on the localization of HA-PPARγ2 and mCherry-Tet1 in the nucleus of NIH/3T3 cells. The inset left below of each image shows the magnified image of the framed area. The graph at the right of each row indicates the transition of the signal intensity of PPARγ2 (green) and Tet1 (red) along with the white allow in the merged image. White bars in the merged images indicate 5 μm. ( b ) Effects of inhibition of PARylation on the interaction of PPARγ with Tet1. HA-PPARγ2 and Myc-Tet1 were transfected to HEK293 cells and immunoprecipitated using anti-HA antibody in the presence or absence of 20 μM PJ-34. Immunoprecipitated HA-PPARγ2 and co-immunoprecipitated Myc-Tet1 was detected by western blotting using anti-PPARγ and anti-Myc antibody. ( c ) PAR-binding assay of Tet1. One microgram of the indicated proteins was dot blotted onto a nitrocellulose membrane and incubated with PAR polymers. Protein-bound polymers were visualized by chemiluminescence with an anti-PAR antibody. pro. K, proteinase K (negative control); Tet1, catalytic domain of Tet1; H1, histone H1 (positive control). ( d ) PAR-binding motifs in Tet1- and PAR-binding assay of Tet1 peptides. (Upper) The schematic depicts the positions of the three putative PAR-binding motifs (m1–3) and four peptides synthesized for the PAR-binding assay (p1-4) of Tet1. Alignment of the putative PAR-binding motifs with the consensus PAR-binding motif is shown below. A common feature of the motif is the presence of hydrophobic amino acids (h; ACGVILMFYW) spaced by basic amino acids (b; KRH) and an additional accumulation of basic residues at the N-terminal side of the motif. Conserved hydrophobic residues are indicated in bold against a red background, and neighbouring basic amino acids are shown in bold against a blue background. The residues corresponding to the basic block of the N-terminal region are represented against a blue background. (Lower) Images of the peptides dyed by CBB and PAR-binding assay of the peptides transferred onto membrane. Full size image To investigate the binding ability of Tet2, we performed a sequence comparison of Tet1 and Tet2 and found that two PAR-binding motifs in Cys-rich domain (m2 and m3) are well conserved in Tet2 ( Supplementary Fig. S19 ). We also found that amino-acid sequences of N-terminals of the two proteins are completely different and Tet2 lacks the m1 motif. PAR-binding assay using Cys-rich domain of Tet2 (Tet2-p3) showed that Tet2-p3 also binds to PAR polymer with almost the same affinity as Tet1-p3. This result suggests that Tet2 also has a potential to bind to PAR polymer and may be recruited to PPRE to contribute to 5hmC production, although we could not experimentally detect the interaction of Tet2 and PPARg by co-IP. These results collectively suggest that the PARylated PPARγ complex attracts Tet1, and probably Tet2, onto the PPRE and triggers the formation of 5hmC. In this study, we have demonstrated that PPARγ directs DNA demethylation around PPREs during differentiation. We have yet to examine the PPREs of other genes expressed in adipocytes; however, we anticipate that they will be demethylated in the same fashion. Our analyses show that the demethylation is mediated by the production of 5hmC around the PPREs, and Tet1 and Tet2 are responsible for it. Other groups have reported that Tet1 and Tet2 have compensatory roles, as knockout and knockdown of Tet1 or Tet2 results in only a partial decrease in 5hmC levels [28] , [31] . Our results also support this observation. Tet1 and Tet2 might have complementary roles to demethylate specific cytosines during the adipocyte differentiation. The DNA demethylation we have observed in this study is a gradual, slow process that takes ~10 days to complete. On the other hand, Kangaspeska et al. [32] observed more rapid demethylation mediated by another nuclear receptor, oestrogen receptor-α. They reported cyclical methylation/demehylation of oestrogen-responsive genes after addition of oestorogen with a periodicity of 100 min. Thillainadesan et al. [33] also reported a rapid demethylation by transforming growth factor-β/SMAD that occurs within 6 h after stimulation. We replicated the experimental conditions used in these reports in our experimental system to check the existence of rapid demethylation in adipogenesis. However, we could not observe any rapid effect like the report ( Supplementary Fig. S20 ). It is probably because the expression level of PPARγ that identifies sites to demethylate is the rate-limiting factor of the demethylation, as suggested in Supplementary Fig. S2 , or underlying mechanism is fundamentally different from these reports. However, we cannot rule out the possibility that other indirect mechanisms may be involved. In this study, all the experiments were done using cultured cell lines. We also measured methylation statuses of Plin1 PPRE in mouse adipose tissues to establish the generality of our report. We collected subcutaneous/visceral adipose tissues and purified genomic DNA of floating adipocyte fraction and stromal vascular fraction (SVF), respectively ( Supplementary Fig. S21 ). RE assay showed that Plin1 PPRE tend to be somewhat demethylated in cells derived from both adipocyte fraction and SVF. It was previously reported that adipogenic promoters are already demethylated at the stage of stromal vascular adipose stem cells, and of course, also in differentiated adipocytes. They also reported that non-adipogenic cells exhibit hypermethylation of these promoters [34] , [35] . Our observation also shows methylated Plin1 PPRE in non-adipogenic cells. The authors concluded in the papers that these promoters are demethylated because adipose stem cells in SVF are already epigenetically committed to adipogenic differentiation. Similarly, we think that Plin1 PPRE, an adipogenic enhancer, is already demethylated in SVF probably because of the same reason. These data suggested that the methylation of PPRE is differently controlled between adipogenic and non-adipogenic cells also in vivo . We found that protein PARylation has a role in PPARγ-driven demethylation around PPREs. To date, we have not been able to determine exactly which protein is PARylated on PPREs, but various proteins included in PPARγ complex are known to be potential targets for PARylation. A previous study reported that PPARγ is itself PARylated by PARP-1 that is involved in the PPARγ complex, which regulates its transcriptional activity [15] . PARP-2 has also been demonstrated to be involved in the PPAR complex on PPREs [14] . Both PARP-1 and PARP-2 are known to PARylate various histones. PARylation of high mobility group proteins and histones lead to a looser chromatin structure at transcription initiation. PARPs are also autoPARylated for the recruitment of other proteins [9] , [36] . More studies are needed to identify the specific target protein for PARylation on PPREs. We have demonstrated in this study that PARylation is associated with the local production of 5hmC during demethylation. Although there are previous reports linking PARylation to DNA demethylation, these suggested that PARylation functioned in the renewal of 5hmC or following intermediate products to unmethylated cytosines by base excision repair. In addition, our findings demonstrated that PARylation of a sequence-dependent transcription factor complex also serves for recruitment of Tet protein and directs the production of 5hmC, thereby inducing localized DNA demethylation. Cell culture 3T3-L1 preadipocytes (JCRB, Japanese Collection of Research Biosources) were cultured in DMEM+10% CS (Gibco Invitrogen) and induced to differentiate into adipocytes using differentiation medium I (DMEM+10% FCS supplemented with 10 μg ml −1 insulin (Sigma), 0.5 mM 3-isobutyl-1-methylxanthine (Sigma) and 1 μM dexamethasone (Sigma)) and II (DMEM+10% FCS supplemented with 5 μg ml −1 insulin). NIH/3T3 and HEK293 cells (JCRB) were cultured in DMEM+10% FCS. Plat-E cells were cultured in DMEM+10% FCS, 10 μg ml −1 blasticidin (Sigma) and 1 μg ml −1 puromycin (Sigma). All cell types were maintained at 37 °C in humidified air with 5% CO 2 . Lentivirus infection Lentivirus infections were performed with the lentivirus expression system provided by RIKEN Bio Resource Center. HEK293 cells were transfected with an expression lentiviral plasmid (Flag-tagged mouse PPARγ2/CSII-EF-MCS-IRES2-Venus, shControl or shTET1-3/CS-RFA-EG) together with a packaging (pCAG-HIVgp) and a VSV-G/Rev-expressing (pCMV-VSV-G-RSV-Rev) plasmid. Thirty-six hours after transfection, the medium containing the lentiviruses was collected and filtered. 3T3-L1 and NIH/3T3 cells were infected with the collected medium (supplemented with 20 μg ml −1 polybrene) for 90 min. The medium was then changed to a fresh culture medium. Retrovirus infection and proviral demethylation assay Retrovirus infections were performed with the Platinum retrovirus expression system (Cell Biolabs). The mouse Plin1 promoter (−3 kbp~transcription start site (TSS)) was cloned into pMXs-IRES-GFP (the primers used for the cloning are listed in Supplementary Table S1 ). To prevent amplification of the endogenous Plin1 promoter in the downstream bisulphite PCR experiments, a point mutation was introduced into the ApaLI site of the cloned promoter to endow ApaLI resistance. Plat-E cells were transfected with this retroviral plasmid and, 48 h after transfection, the culture medium containing retroviruses was collected and filtered. 3T3-L1 and NIH/3T3 cells were infected with the medium (supplemented with 20 μg ml −1 polybrene) for 6 h. The medium was then removed and replaced with fresh medium. The cells were subcultured on days 4 and 8, and were induced to differentiate (3T3-L1) or were infected with PPARγ lentivirus (NIH/3T3) on day 10. Total genomic DNA was collected at the indicated time points and completely digested with ApaL1 before being used as a template for bisulphite conversion. Bisulphite PCR and RE digestion assays were performed as described in the pertinent section. Determination of DNA methylation status by bisulphite conversion Bisulphite treatment of genomic DNA was carried out using EZ DNA Methylation-Gold Kit (Zymo Research) in accordance with the manufacturer’s instructions. Regions of interest were then amplified by PCR using the primers listed in Supplementary Table S1 . For bisulphite sequencing, PCR fragments were cloned with pGEM T-Easy vector system (Promega) and 10 clones were sequenced to determine the methylation status. For the RE digestion assay, the region around the digestion site of the Plin1 promoter was PCR amplified with the primers listed in Supplementary Table S1 . The amplified fragments were digested with HpyCH4IV (New England Biolabs) that cuts at ‘ACGT’. Completely reacted fragments were electrophoresed to separate the digested (that is, methylated: ACGT) fragments and undigested (that is, unmethylated: ATGT) fragments. The proportions of digested and undigested fragments were calculated from ethidium bromide-stained agarose gel images using ImageJ 1.42q (NIH). Quantification of 5hmC by dot blot analysis Purified genomic DNA was heat-denatured at 95 °C for 10 min, and chilled on ice for 1 min. One hundred nanograms of the DNA were spotted onto a piece of Hybond-N+ membrane (Amersham) and then ultraviolet crosslinked. The membranes were blocked with 5% skim milk in TBS, and then signals were detected using an anti-5hmC antibody (Active motif) and horseradish peroxidase-conjugated secondary antibodies. Analyses of mRNA expressions by reverse transcriptase–PCR Total RNA was extracted using an RNeasy Mini Kit (Qiagen) and was converted into first-strand complementary DNA by synthesis with random hexamers using a Transcriptor First Strand cDNA Synthesis Kit (Roche). The synthesized cDNA was used as the template for PCR amplification of Plin1 , PPARγ and β-actin. The primers used for amplification are listed in Supplementary Table S1 . For Plin1 and PPARγ, the PCR reactions were performed using the following conditions: 95 °C, 2 min; 30 cycles of 95 °C, 10 s; 55 °C, 10 s; 72 °C, 10 s. For β-actin, the following conditions were used: 95 °C, 2 min; 25 cycles of 95 °C, 10 s; 55 °C, 10 s; 72 °C, 10 s. Chromatin immunoprecipitation assay NIH/3T3 cells expressing FLAG-PPARγ2 (day 5, treated with or without 20 μM PJ-34) were crosslinked by formaldehyde and sonicated on ice. DNA–protein complexes were immunoprecipitated using an anti-PAR polymer antibody (Trevigen) or anti-FLAG antibody (Sigma). The amount of DNA containing a demethylated region around the PPRE and unrelated control region were quantified by PCR. The following PCR conditions were used: 95 °C, 2 min; 30 cycles of 95 °C, 10 s; 55 °C, 10 s; 72 °C, 10 s. Primers used for the amplification are listed in Supplementary Table S1 . One percent of the input was set aside before immunoprecipitation and amplified using the same conditions. Immunofluorescence microscopy NIH/3T3 cells were grown on glass coverslips and co-transfected with PPARγ2/pCMV-HA and Tet1 (a.a. 1367–2039)/pmCherry-C1 constructs a day before fixation. Cells were then fixed and permeabilized with MeOH/acetone (1/1, v/v) for 10 min at 4 °C. Cells were incubated with primary antibodies (anti-HA, Roche (1:1000); anti-PAR, Trevigen (1:250)) diluted in 5% skim milk in PBS for 2 h. After incubation with Alexa Fluor 488 (Molecular Probes (1:1000)) or Cy3-conjugated secondary antibodies (Chemicon (1:1000)) diluted in 5% skim milk in PBS, images were acquired with a confocal microscope LSM710 (Carl Zeiss) and analysed by Zeiss Efficient Navigation (Carl Zeiss). Immunoprecipitation assay Nuclear extracts were prepared from 3T3-L1 cells (day 5) or HEK293 cells expressing HA-PPARγ2 and Myc-Tet1, and were diluted with IP buffer (50 mM Tris–HCl (pH 8.0), 100 mM NaCl, 5 mM MgCl2, 0.2% NP-40). Antibodies were incubated with Dynabeads protein A (Life Technologies) in advance and added to the diluted nuclear extract. After an overnight incubation, the beads were washed with IP buffer and the immunoprecipitated proteins were analysed by western blotting. The antibodies used were as follows: anti-PPARγ (Perseus Proteomics), anti-Tet1 (Millipore), anti-HA tag (Cell Signaling) and anti-Myc tag (MBL). Antibodies were used in the amount of 5 μg per IP. DNA immunoprecipitation assay Ten micrograms of genomic DNA from PPARγ2-expressing NIH/3T3 (day 5) were digested with Mse I and Xba I. The digested sample was heat-inactivated at 65 °C for 15 min, and diluted with 10 mM Tris–HCl (pH 8.0), 1 mM EDTA, 140 mM NaCl, 0.05% Triton-X100. Fragments containing 5hmC or 5mC were then immunoprecipitated using 1 μg of an anti-5hmC antibody (Active Motif) or 3 μg of an anti-5mC antibody (Active Motif), and the DNA fragments containing the demethylated region or the control region were quantified by real-time PCR (Applied Biosystems, 7500 Real Time PCR System; Nippon Genetics, KAPA SYBR FAST qPCR kit). The control region was selected to contain a similar number of CpGs as the demethylated region of each gene: for Plin1 , nine CpGs in both the control and demethylated regions; for aP2 , seven CpGs in the control region and eight CpGs in the demethylated region. The primers used for the amplification are listed in Supplementary Table S1 . Five percent of the input was set aside before immunoprecipitation and estimated using the same conditions. Poly (ADP-ribose)-binding assay For dot blot analyses, 1 μg of each protein was blotted onto a strip of nitrocellulose membrane. For analyses of Tet peptides, 500 ng of each recombinant peptide was separated by polyacrylamide gel electrophoresis and transferred onto nitrocellulose membrane. The membrane was briefly washed with TBS containing 0.05% (v/v) Tween 20 (TBST) and incubated with PAR polymers (50 nM in TBST; Trevigen). After incubation for 1 h at room temperature, unbound PAR polymers were washed off with TBST, and the membranes were blocked with 5% skim milk in TBST. The protein-bound PAR polymers were then detected with an anti-PAR polymer antibody (Trevigen) and horseradish peroxidase-conjugated secondary antibody, and were visualized by Western Lightning Plus-ECL (PerkinElmer). The following purified proteins were purchased from each manufacturer: Tet1 (a.a. 1367–2039), Active Motif; Histone H10, (New England Biolabs); proteinase K, Takara. Tet1 peptides p1-4 and Tet2-p3 were synthesized in bacteria with the pET-15b vector system (Novagen) and purified with the MagneHis Protein Purification System (Promega). Tet peptides, respectively, correspond to the regions of amino-acid residues of Tet1 as follows: Tet1-p1, a.a.1–200; Tet1-p2, a.a.483–687; Tet1-p3, a.a.1272–1621; Tet1-p4, a.a.1626–1975; Tet2-p3, a.a. 959–1264. How to cite this article: Fujiki, K. et al. PPARγ-induced PARylation promotes local DNA demethylation by production of 5-hydroxymethylcytosine. Nat. Commun. 4:2262 doi: 10.1038/ncomms3262 (2013).